Delivery of chemotherapeutic drugs in tumour cell-derived microparticles Cellular microparticles are vesicular plasma membrane fragments with a diameter of 100–1,000 nanometres that are shed by cells in response to various physiological and artificial stimuli. Here we demonstrate that tumour cell-derived microparticles can be used as vectors to deliver chemotherapeutic drugs. We show that tumour cells incubated with chemotherapeutic drugs package these drugs into microparticles, which can be collected and used to effectively kill tumour cells in murine tumour models without typical side effects. We describe several mechanisms involved in this process, including uptake of drug-containing microparticles by tumour cells, synthesis of additional drug-packaging microparticles by these cells that contribute to the cytotoxic effect and the inhibition of drug efflux from tumour cells. This study highlights a novel drug delivery strategy with potential clinical application. The selective delivery of chemotherapeutic drugs to tumour cells is a major challenge in cancer chemotherapy. Recent studies show that packaging clinically approved drugs into nanoscale vesicular vehicles (10–100 nm in diameter) can effectively deliver chemotherapeutic drugs to tumour sites, leading to improved pharmacokinetic efficiency and therapeutic efficacy [1] , [2] . Nonetheless, these drug-loaded artificial nanoparticles have several disadvantages. First, nanometre-scale materials, as nonself components, are usually toxic and may cause adverse effects, for example, by activating oxidative stress pathways [2] , [3] , [4] , [5] , [6] , [7] ; second, micelles are of inadequate stability in the blood stream; third, co-encapsulation of more than one drug can result in batch-to-batch variability in the drug load; and fourth, the cost of assembly of nanoparticles is expensive, especially if they contain engineered antibodies or aptamers. Notwithstanding these defects, the development of advanced nanoparticle drug carriers is currently vigorously pursued in the field of cancer therapeutics [1] , [7] . However, one facet or direction, often overlooked, is the existence and efficacy of natural counterparts to these artificial nanoparticles. Cells are capable of generating various vesicles of different sizes but whether these cell-derived microvesicles are suitable for drug delivery remains unclear. In response to various stimuli, cells may change their cytoskeletal structure and result in the encapsulation of cytosolic elements by the plasma membrane that are then released into the extracellular space. These specialized subcellular vesicles with a diameter of 100–1,000 nm are called microparticles (MPs) [8] , [9] . Wolf first observed MPs from activated blood platelets in 1967 and described them as pro-coagulant ‘dust’ [10] . Since then, it has progressively become more evident that MPs can be derived from almost all cell types and have crucial roles under physiological or pathophysiological conditions [8] , [11] . MPs not only contain messenger molecules, enzymes, RNAs and even DNA, but also are capable of transferring these bioactive molecules from one cell to another [12] , [13] , [14] , [15] . Thus, functionally, MPs appear to act as vectors delivering molecular messages between cells. Considering these similarities of MPs with nanoparticles in size, structure and vector function, it is reasonable to hypothesize that MPs may be useful as endogenous natural vehicles to deliver chemotherapeutic drugs. This study demonstrates that MPs, derived from apoptotic tumour cells, can package and deliver chemotherapeutic drugs to tumour cells, thereby, leading to the timely death of the tumour cells without typical drug-associated side effects. Development of tumour cell-derived drug-encapsulating MPs We first tested whether apoptotic tumour cells, induced by chemotherapeutic drugs, could produce drug packaging MPs. For this purpose, carboxyfluorescein succinimidyl ester (CFSE)-stained mouse hepatocarcinoma tumour cell line H22 were incubated with 10 μg ml −1 methotrexate (MTX) and then irradiated with ultraviolet light for further apoptosis induction. The MPs were isolated [16] , [17] , and analysed by flow cytometry. Apoptotic tumour cells could indeed release considerable MPs ( Fig. 1a , left). As large as 3 × 10 5 MPs were yielded from 5 × 10 6 tumour cells ( Fig. 1a , right). These MPs were not generated owing to background noise or nonspecific events ( Supplementary Fig. S1 ), and showed membrane structures with 100–1,000-nm sizes as judged by electron microscopy ( Fig. 1b ). Such membrane structures were further confirmed by western blot ( Supplementary Fig. S2 ) and by flow cytometric analysis of MPs derived from Raw 264.7 cells ( Supplementary Fig. S3 ). Given the fluorescent nature of doxorubicin [18] , we employed doxorubicin fluorescence to determine whether the drug is packaged into the released MPs. Doxorubicin was clearly shown to be encapsulated by MPs ( Fig. 1c ). Moreover, high-performance liquid chromatography (HPLC) analysis showed that the different concentrations of doxorubicin or MTX in MPs were owing to drug doses ( Fig. 1d , Supplementary Fig. S4 ). Besides H22 cells, the human ovarian cancer tumour cell line A2780 also produced MPs after the treatment by cisplatin ( Fig. 1a ) or doxorubicin ( Fig. 1c ), suggesting that tumour cells may indeed generate drug-encapsulating MPs in response to chemotherapeutic treatments. 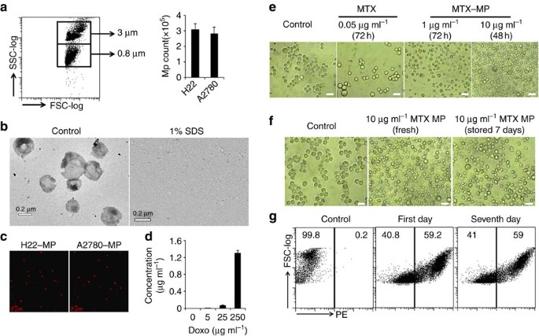Figure 1: MPs are cytotoxic after encapsulating chemotherapeutic drugs. (a) Apoptotic tumour cells released a large number of MPs. CFSE-labelled H22 cells (5 × 106) were incubated with 10 μg ml−1MTX and irradiated with ultraviolet B. After 12 h, MPs were isolated and counted by a flow cytometer on the basis of 0.8 μm beads (left). Data are the representative of three independent experiments. Bars correspond to mean±s.d. (b) MPs treated with or without 1% SDS were analysed by transmission electron microscope. (c) Tumour cells treated with chemotherapeutic drugs released drug-packaging MPs. H22 cells or A2780 cells were incubated with 100 μg ml−1doxorubicin and irradiated with UBV. MPs were isolated and observed under two-photon laser scanning fluorescence microscope. Doxorubicin was shown as the red colour. Scale bar, 2 μm. (d) The concentration of doxorubicin in MPs was measured by HPLC. Data are the representative of three independent experiments. Bars correspond to mean±s.d. (e) Drug-encapsulating MPs were cytotoxic to tumour cells. MTX (1 or 10 μg ml−1) was added to H22 tumour cells (5 × 106) for 1 h and then treated with UBV. After isolation 12 h later, half of MTX-encapsulating MPs were incubated with H22 tumour cells. The death of tumour cells was observed at different time points. H22 cells treated with 0.05 μg ml−1MTX were observed after 72 h. Scale bar, 25 μm. (f,g) Chemotherapeutic drug-encapsulating MPs were stable. MPs from MTX-treated H22 tumour cells were stored at 4 °C for 7 days, and then added to H22 cell culture medium for cytotoxicity assay. Scale bar, 25 μm (f). MPs from doxorubicin-treated H22 cells or untreated cells as control were stored at 4 °C for 7 days and the stability of these MPs was analysed by flow cytometry (g). MPs without doxorubicin served as control and doxorubicin-packaging MPs were reflected by the positive dot plots. In this figure, 10,000–20,000 events were collected for flow cytometric analysis. Figure 1: MPs are cytotoxic after encapsulating chemotherapeutic drugs. ( a ) Apoptotic tumour cells released a large number of MPs. CFSE-labelled H22 cells (5 × 10 6 ) were incubated with 10 μg ml −1 MTX and irradiated with ultraviolet B. After 12 h, MPs were isolated and counted by a flow cytometer on the basis of 0.8 μm beads (left). Data are the representative of three independent experiments. Bars correspond to mean±s.d. ( b ) MPs treated with or without 1% SDS were analysed by transmission electron microscope. ( c ) Tumour cells treated with chemotherapeutic drugs released drug-packaging MPs. H22 cells or A2780 cells were incubated with 100 μg ml −1 doxorubicin and irradiated with UBV. MPs were isolated and observed under two-photon laser scanning fluorescence microscope. Doxorubicin was shown as the red colour. Scale bar, 2 μm. ( d ) The concentration of doxorubicin in MPs was measured by HPLC. Data are the representative of three independent experiments. Bars correspond to mean±s.d. ( e ) Drug-encapsulating MPs were cytotoxic to tumour cells. MTX (1 or 10 μg ml −1 ) was added to H22 tumour cells (5 × 10 6 ) for 1 h and then treated with UBV. After isolation 12 h later, half of MTX-encapsulating MPs were incubated with H22 tumour cells. The death of tumour cells was observed at different time points. H22 cells treated with 0.05 μg ml −1 MTX were observed after 72 h. Scale bar, 25 μm. ( f , g ) Chemotherapeutic drug-encapsulating MPs were stable. MPs from MTX-treated H22 tumour cells were stored at 4 °C for 7 days, and then added to H22 cell culture medium for cytotoxicity assay. Scale bar, 25 μm ( f ). MPs from doxorubicin-treated H22 cells or untreated cells as control were stored at 4 °C for 7 days and the stability of these MPs was analysed by flow cytometry ( g ). MPs without doxorubicin served as control and doxorubicin-packaging MPs were reflected by the positive dot plots. In this figure, 10,000–20,000 events were collected for flow cytometric analysis. Full size image Tumour cell-derived drug-encapsulating MPs are cytotoxic To verify whether drug-encapsulating MPs are cytotoxic to tumour cells, low or high concentrations of MTX (1 or 10 μg ml −1 ) were added to the cultured H22 cells (5 × 10 6 ) 1 h before ultraviolet irradiation. After 12 h, the released MTX-encapsulating MPs were incubated with H22 cells. Both high and low concentrations of MTX–MPs could induce tumour cell death after 48 or 72 h ( Fig. 1e , Supplementary Fig. S5 ). Consistently, the higher drug dosage resulted in MP packaging more drug molecules. MPs from 100 μg ml −1 doxorubicin-treated H22 cells showed much stronger mean fluorescence intensity (MFI) than that from 10 μg ml −1 doxorubicin-treated H22 cells (1,316 versus 623). In addition, other drugs, such as cisplatin and hydroxyl camptothecin, and other cell lines, including A2780, B16, HL60 and EL4, were also tested, and the generated drug-packaging MPs also resulted in the similar results. Interestingly, the addition of MPs, generated from 1 μg MTX-treated H22 tumour cells, cultured in 1 ml medium, resulted in obviously discernible tumour cell killing, whereas the addition of 0.05 μg MTX to the same culture media had no discernible cytotoxic effect ( Fig. 1e , Supplementary Fig. S5 ). Furthermore, 0.6 μg MTX only killed around 2% H22 tumour cells in a 1 ml medium, whereas MPs packaging 0.6 μg MTX (based on HPLC results) induced around 23% tumour cell death ( Supplementary Fig. S6 ), suggesting that tumour cell-derived drug-encapsulating MPs might have a higher tumour-killing efficacy or efficiency than conventional chemotherapeutic drugs. To further assess this pharmacological efficacy, the stability of MPs was tested. We found that doxorubicin-encapsulating MPs were at least stable for 1 week at 4 °C ( Fig. 1f ), and such stored MPs possessed a similar capability to kill H22 cells ( Fig. 1e ). In addition, MPs were found to be resistant to acidic and alkaline environments, light, shaking and high temperatures (room temperature or 37 °C), but not to SDS or proteinase K ( Supplementary Fig. S7 ). As MPs were generated from apoptotic tumour cells, we also analysed cell death molecules by using western blot or DNA gel. Consistent with the previous report [19] , we found that MPs contained a panel of natural biomolecules, such as cytochrome c, caspases 3 and 9, histones and DNA pieces ( Supplementary Fig. S8 ). Together, these findings demonstrated that tumour cell-derived MPs are indeed capable of encapsulating chemotherapeutic drug, are cytotoxic to tumour cells and more effective than direct treatment with the same drug on a dose-per-dose basis. MTX-encapsulating MPs inhibit ascites hepatocarcinoma growth To address whether MPs could be used for anticancer therapy in vivo , we injected MTX-encapsulating MPs intravenously (i.v.) or intraperitoneally (i.p.) into mice. Two milligram MTX were added to 2 ml culture media with 2 × 10 7 H22 tumour cells 1 h before ultraviolet irradiation. Each of the prepared MPs was then used for one mouse per package. Collectively, mice were treated once per day for 6 days. Compared with simple MPs or PBS control, MTX–MPs did not induce any hair and/or weight changes in the mice or adversely affect liver or kidney functions ( Fig. 2a ). In contrast, twice repeated i.v. or i.p. injections of 2 μg g −1 MTX produced typical side effects ( Fig. 2a ). We then assessed the therapeutic efficacy of MTX-packaging MPs in a murine hepatocarcinoma ascites model. The i.p. injection of H22 cells formed obvious ascites within 10 days. The next day after the i.p. tumour cell inoculation, the mice were given treatments of MPs once per day for 5 days. On day 10, the mice were killed and the volume of ascites measured. The results showed that the volume of ascites was significantly reduced in the mice treated with MTX–MPs compared with control groups ( Fig. 2b ). Consistently, MTX–MPs-treated mice had much longer survival time ( Fig. 2c ), clearly suggesting that MTX-encapsulating MPs inhibit tumour growth without typical side effects in a murine hepatocarcinoma ascites model. 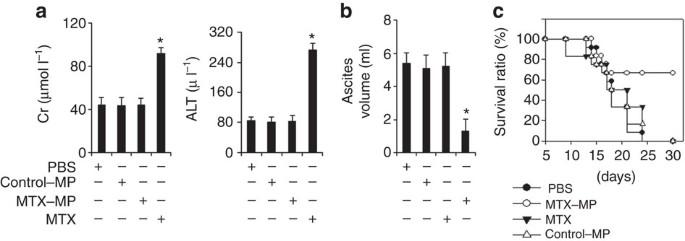Figure 2: MTX-packaging MPs inhibit peritoneal H22 cell growth without typical side effects. (a) MTX-encapsulating MPs did not adversely impact liver or kidney functions. 2 × 107H22 cells were incubated with 2 mg MTX in 2 ml culture medium for 1 h before ultraviolet irradiation, and the isolated MPs were injected i.v. or i.p. to one mouse once per day for 6 days (n=8 for each group). Serum levels of glutamic-pyruvate transaminase and creatinine were detected. MPs from sole UBV-treated H22 cells and the two time injection of 2 μg g−1MTX were used as controls. Bars correspond to mean±s.d. The data shown were representative of three reproducible experiments. (b,c) MTX–MPs inhibited tumour growth. H22 cells were i.p. injected mice (n=12 for each group). On day 1, MPs from 1 mg ml−1MTX-treated H22 cells or UBV-treated cells were i.p. injected to the mice once per day for 10 days. Or, single MTX (0.5 μg g−1) was i.p. injected to mice once per day for 5 days. On day 11, half the mice in each group were killed and the volume of ascites was measured (b). The rest of the mice were used for long-term survival observation (c). Data are representative of three independent experiments.P<0.001, MTX.MP group compared with PBS control group. Figure 2: MTX-packaging MPs inhibit peritoneal H22 cell growth without typical side effects. ( a ) MTX-encapsulating MPs did not adversely impact liver or kidney functions. 2 × 10 7 H22 cells were incubated with 2 mg MTX in 2 ml culture medium for 1 h before ultraviolet irradiation, and the isolated MPs were injected i.v. or i.p. to one mouse once per day for 6 days ( n =8 for each group). Serum levels of glutamic-pyruvate transaminase and creatinine were detected. MPs from sole UBV-treated H22 cells and the two time injection of 2 μg g −1 MTX were used as controls. Bars correspond to mean±s.d. The data shown were representative of three reproducible experiments. ( b , c ) MTX–MPs inhibited tumour growth. H22 cells were i.p. injected mice ( n =12 for each group). On day 1, MPs from 1 mg ml −1 MTX-treated H22 cells or UBV-treated cells were i.p. injected to the mice once per day for 10 days. Or, single MTX (0.5 μg g −1 ) was i.p. injected to mice once per day for 5 days. On day 11, half the mice in each group were killed and the volume of ascites was measured ( b ). The rest of the mice were used for long-term survival observation ( c ). Data are representative of three independent experiments. P <0.001, MTX.MP group compared with PBS control group. Full size image Cisplatin-encapsulating MPs inhibit ovarian cancer growth To further confirm that tumour cell-derived chemotherapeutic drug-encapsulating MPs have an anticancer activity, human ovarian cancer in severe combined immunodeficient (SCID) mice was also tested by i.p. injection of A2780 cells. Six hundred micrograms cisplatin was added to 2-ml culture media with 2 × 10 7 A2780 cells 1 h before ultraviolet irradiation. The MPs formed were then used for one mouse each. Similar to the above MTX–MPs, the administration of cisplatin–MPs continuously for 5 days did not affect liver and kidney functions of SCID mice either. In order to test their therapeutic efficacy, cisplatin–MPs were administered to mice 5 days after A2780 cell inoculation. After 14 days, an additional treatment was administered once per day for 5 days. After 30 days, SCID mice were killed and the tumour growth evaluated. As shown in Fig. 3a , almost no tumour nodes were observed in the cisplatin–MP group. In contrast, a large number of tumour nodes was seen in control–MP group. Consistently, cisplatin–MP-treated mice had much longer survival times ( Fig. 3b ). Moreover, MPs packaging cisplatin and paclitaxel almost completely suppressed A2780 tumour growth in nude mice ( Supplementary Fig. S9 ). Therefore, A2780 cell-derived MPs inhibit human ovarian cancer growth in SCID mice by packaging cisplatin or cisplatin/paclitaxel. 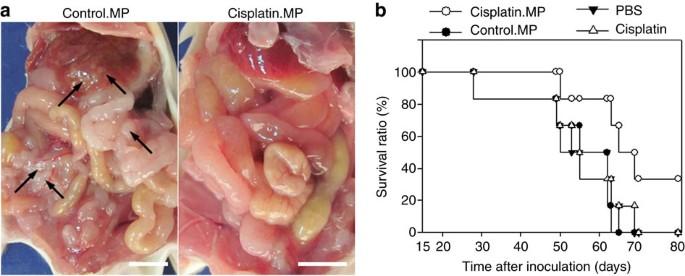Figure 3: Cisplatin-packaging MPs inhibit ovarian cancer growth in SCID mice. (a,b) A2780 cells were i.p. injected to SCID mice (n=12 per group). From the next day, mouse was administered with MPs or with single cisplatin (2 μg g−1) or PBS by i.p. injection once per day for continuous 5 days. After 14 days, an additional treatment was administered once per day for 5 days. After 30 days, half the mice were killed and the tumour nodes were observed. The typical nodes were shown by the arrow. Scale bar, 1 cm. (a). The remaining mice were used for the long-term survival observation (b). Data are representative of three independent experiments.P<0.001, Cisplatin.MP group compared with PBS control group. Figure 3: Cisplatin-packaging MPs inhibit ovarian cancer growth in SCID mice. ( a , b ) A2780 cells were i.p. injected to SCID mice ( n =12 per group). From the next day, mouse was administered with MPs or with single cisplatin (2 μg g −1 ) or PBS by i.p. injection once per day for continuous 5 days. After 14 days, an additional treatment was administered once per day for 5 days. After 30 days, half the mice were killed and the tumour nodes were observed. The typical nodes were shown by the arrow. Scale bar, 1 cm. ( a ). The remaining mice were used for the long-term survival observation ( b ). Data are representative of three independent experiments. P <0.001, Cisplatin.MP group compared with PBS control group. Full size image Tumour cells take up chemotherapeutic drug-packaging MPs To elucidate the mechanism by which drug-encapsulating MPs efficiently mediate tumour cell killing, we first asked whether the interaction between MPs and tumour cells were required for tumour cell killing. MTX–MPs were incubated in culture media for 48 h and separated from the media by centrifugation. Interestingly, only the separated MTX–MPs, but not the corresponding supernatants or the supernatants from the last MPs washing, were cytotoxic ( Fig. 4a ), suggesting that chemotherapeutic drugs are within and not discharged from MPs. This was in line with the previous result of Fig. 1d , which showed that MPs were very stable. Here, it was further observed that MPs were Triton X-100 resistant ( Fig. 4b , Supplementary Fig. S7 ), hinting a direct interaction between tumour cells and MPs. In addition, MPs derived from CFSE-stained H22 cells were incubated with PKH26-stained H22 cells. It was found that the green MPs were efficiently taken up by red H22 cells ( Fig. 4c ) and around 54% H22 cells took up MPs ( Fig. 4d ). To test this result in vivo , doxorubicin-packaging MPs were i.p. injected into mice that previously received an injection of H22 cells. About 11.8% of the tumour cells were found red fluorescent and most of these red cells could be stained with Annexin V, the marker of cellular apoptosis ( Fig. 4e ). In parallel, after the injection of MTX-packaging MPs to mice peritoneal H22 tumour for 5 days, peritoneal immune cells were isolated for apoptotic analysis. As shown in Fig. 4f , drug-packaging MPs effectively induced the apoptosis of F4/80 + macrophages but had no effect on CD3 + T or CD19 + B cells. Consistently, H22 MPs were strongly taken up by H22 cells, but not by T or B cells in vitro ( Supplementary Fig. S10a,b ). As H22 cells are hepatocyte derived, primary liver cells were additionally assessed to take up MPs. It was found that the drug-packaging MPs were weakly taken up by and had minor effect on the primary liver cells ( Supplementary Fig. S11a,b ), suggesting that MPs are efficiently taken up by tumour cells. 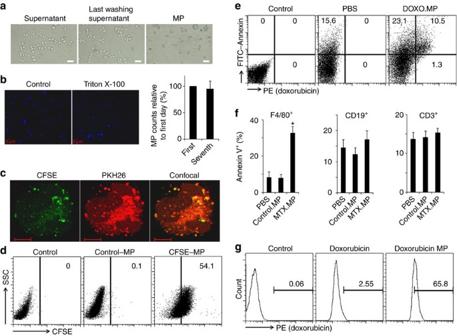Figure 4: MPs efficiently deliver chemotherapeutic drug molecules into tumour cells. (a) H22 cells were treated with 100 μg MTX. After separation by centrifugation, MTX–MPs, the corresponding supernatants or the supernatants from the last MPs washing were co-cultured with H22 cells. After 48 h, the tumour cell killing was observed. Scale bar, 25 μm. (b) MPs were resistant to Triton X-100. MPs from H22 cells were treated with or without 0.5% Triton X-100 for 12 h and then incubated with Hoechst 33342. After 12 h, MPs were isolated for the observation under a fluorescence microscope (left) or counted by a flow cytometer (right). Bars correspond to mean±s.d. Data are representative of three independent experiments. Scale bar, 2 μm. (c,d) H22 cells took up MPs. MPs isolated from CFSE (green)-labelled H22 cells were incubated with PKH 26 (red)-stained H22 cells. After 20 h, cells were observed under two-photon laser scanning fluorescence microscope, (c), or analysed by flow cytometry (d). Data are representative of three reproducible independent experiments. Scale bar, 10 μm. (e) Doxorubicin-packaging MPs were i.p. injected into mice, to which H22 cells were i.p. injected 24 h before. Twenty-four hours after MP injection, peritoneal tumour cells were isolated and stained with FITC–Annexin V for flow cytometric analysis. (f) MPs isolated from MTX-treated or -untreated H22 cells were i.p. injected to mice (n=6). After 5 days injection, peritoneal immune cells were isolated and stained with PE-conjugated Annexin V and FITC-conjugated anti-F4/80, CD19 or CD3 antibody. The cells were analysed by flow cytometry. Bars correspond to mean±s.d. *P<0.05, compared with control. (g) MPs improved the delivery efficiency of chemotherapeutic drug to tumour cells. The details were described in the Result part and Methods. In this figure, 10,000 events were collected for flow cytometric analysis. Figure 4: MPs efficiently deliver chemotherapeutic drug molecules into tumour cells. ( a ) H22 cells were treated with 100 μg MTX. After separation by centrifugation, MTX–MPs, the corresponding supernatants or the supernatants from the last MPs washing were co-cultured with H22 cells. After 48 h, the tumour cell killing was observed. Scale bar, 25 μm. ( b ) MPs were resistant to Triton X-100. MPs from H22 cells were treated with or without 0.5% Triton X-100 for 12 h and then incubated with Hoechst 33342. After 12 h, MPs were isolated for the observation under a fluorescence microscope (left) or counted by a flow cytometer (right). Bars correspond to mean±s.d. Data are representative of three independent experiments. Scale bar, 2 μm. ( c , d ) H22 cells took up MPs. MPs isolated from CFSE (green)-labelled H22 cells were incubated with PKH 26 (red)-stained H22 cells. After 20 h, cells were observed under two-photon laser scanning fluorescence microscope, ( c ), or analysed by flow cytometry ( d ). Data are representative of three reproducible independent experiments. Scale bar, 10 μm. ( e ) Doxorubicin-packaging MPs were i.p. injected into mice, to which H22 cells were i.p. injected 24 h before. Twenty-four hours after MP injection, peritoneal tumour cells were isolated and stained with FITC–Annexin V for flow cytometric analysis. ( f ) MPs isolated from MTX-treated or -untreated H22 cells were i.p. injected to mice ( n =6). After 5 days injection, peritoneal immune cells were isolated and stained with PE-conjugated Annexin V and FITC-conjugated anti-F4/80, CD19 or CD3 antibody. The cells were analysed by flow cytometry. Bars correspond to mean±s.d. * P <0.05, compared with control. ( g ) MPs improved the delivery efficiency of chemotherapeutic drug to tumour cells. The details were described in the Result part and Methods. In this figure, 10,000 events were collected for flow cytometric analysis. Full size image Efficiency of MP-mediated drug delivery To clarify whether drugs within MPs are delivered more efficiently to tumour cells than those not packaged into MPs, MPs from 100-μg doxorubicin-treated 1 × 10 7 tumour cells in 4-ml culture media were prepared, and then 10% of the prepared MPs and the corresponding 10 μg doxorubicin were added to 1 × 10 7 tumour cells in 4-ml fresh media, respectively. After 4 h, cells were collected for flow cytometric analysis. In the MP group, tumour cells effectively took up MPs and showed strikingly high fluorescence. In contrast, in the 10-μg doxorubicin group, although tumour cells showed positive fluorescence the relative intensity was much weaker ( Fig. 4g ). To clarify whether MPs have the same efficiency in vivo , doxorubicin-packaging MPs and the same dose-containing doxorubicin as MPs (according to HPLC results) were i.p. injected into mice that previously received an injection of H22 tumour cells. After 12 h, peritoneal tumour cells were isolated and detected by flow cytometry. The result showed that compared with simple drug administration, MPs resulted in an eightfold increase in the delivery efficiency of doxorubicin to tumour cells ( Supplementary Fig. S12 ). Taken together, these data suggest that MPs may concentrate the dispersive chemotherapeutic drug molecules and directly deliver them to tumour cells. Drug-encapsulating MPs induce domino-like tumour cell killing The concentration of drugs in tumour cells may explain why tumour cells were killed by MPs. However, it left unexplained why relatively few MPs could kill many tumour cells, as shown in Fig. 1 . One possibility was that tumour cells killed by MTX–MPs form new MTX-packaging MPs, which are also cytotoxic. To test this hypothesis, H22 cells were incubated with MTX–MPs. After washing, tumour cells were put into new culture media and the new MPs were isolated. As expected, the second generation of MPs also induced H22 tumour cell death ( Fig. 5a ). As additional corroboration, when H22 tumour cells were treated with doxorubicin, it was found that doxorubicin was included in the second generation of MPs ( Fig. 5b ). Moreover, the third generation of MPs still contained the original drug and had cytotoxic activity against H22 cells ( Fig. 5a ). Thus, chemotherapeutic drug-encapsulating MPs may generate a domino-like tumour killing effect. 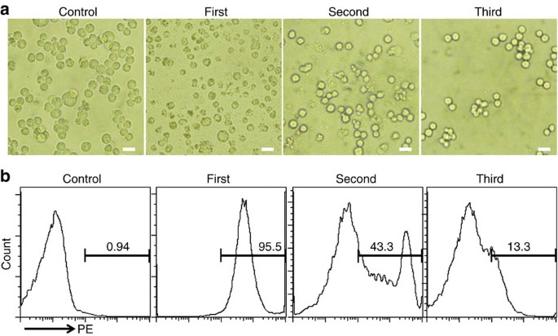Figure 5: Drug-containing MPs induce the formation of additional drug-packaging MPs. (a) MPs isolated from 1 mg ml−1MTX-treated 5 × 107H22 cells were designated as the first generation. These MPs were added to 1 × 107H22 tumour cells and washed out with fresh culture medium 6 h later, from which the generated MPs were called second generation of MPs. In the same way, a third generation of MPs was obtained. These three generations of MTX-packaging MPs were incubated with 1 × 105H22 cells, respectively, for 48 h and the tumour cell death was observed. Scale bar, 25 μm. (b) Red fluorescent intensity of three generations of doxorubicin-packaging MPs was measured by flow cytometry. Ten thousand events were collected for this analysis and data were representative of three reproducible independent experiments. Figure 5: Drug-containing MPs induce the formation of additional drug-packaging MPs. ( a ) MPs isolated from 1 mg ml −1 MTX-treated 5 × 10 7 H22 cells were designated as the first generation. These MPs were added to 1 × 10 7 H22 tumour cells and washed out with fresh culture medium 6 h later, from which the generated MPs were called second generation of MPs. In the same way, a third generation of MPs was obtained. These three generations of MTX-packaging MPs were incubated with 1 × 10 5 H22 cells, respectively, for 48 h and the tumour cell death was observed. Scale bar, 25 μm. ( b ) Red fluorescent intensity of three generations of doxorubicin-packaging MPs was measured by flow cytometry. Ten thousand events were collected for this analysis and data were representative of three reproducible independent experiments. Full size image Tumour cell-derived MPs impede drug efflux To further elucidate MP-mediated killing efficiency, we turned our attention to whether MPs acted as a biomaterial that influences drug-mediated tumour cell killing. MPs were found to be resistant to the effects of Triton X-100 ( Fig. 4b ), suggesting that lipid raft structure is involved in membrane origination of MPs. Interestingly, lipid rafts are known to be connected to drug efflux [20] , [21] , [22] , begging the question whether MPs might influence drug efflux in tumour cells. Therefore, H22 tumour cells were incubated with H22 tumour cell-derived MPs for 12 h, followed by the addition of 0.8 μg ml −1 doxorubicin for 6 h, and then the supernatant was replaced with the fresh medium for another 6-h culture. The drug efflux by tumour cells was then evaluated by flow cytometric analysis of intracellular fluorescent intensity. The results in the form of a decrease of MFI from 1,377 to 593 showed that H22 cells can effectively evacuate doxorubicin within 6 h ( Fig. 6a ). However, MPs strikingly inhibited this decrease by MFI from 1,299 to 1,086 ( Fig. 6a ). Moreover, the simultaneous addition of MPs and doxorubicin also impeded the decrease of MFI from 1,259 to 788 ( Fig. 6a ), suggesting that MPs might prevent the efflux of chemotherapeutic drug by tumour cells. In line with this result, we found that pretreatment of H22 tumour cells by MPs enhanced MTX-induced tumour cell apoptosis ( Fig. 6b ). Therefore, tumour cell-derived MPs were deemed capable of impeding drug efflux, leading to increased tumour cell sensitivity to chemotherapeutic agents. 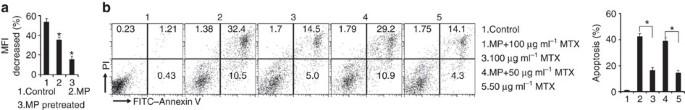Figure 6: MPs enhance tumour cell susceptibility to chemotherapy. (a) MPs decreased the efflux of drugs in H22 cells. H22 tumour cells were incubated with H22 cell-derived MPs for 12 h, then treated with 1 μg ml−1doxorubicin. After 6 h, the supernatant was replaced with the fresh medium for another 6 h culture. The drug efflux by tumour cells was evaluated by flow cytometry and presented as the decrease of MFI. Data were combined from four reproducible experiments. Bars correspond to mean±s.d. (b) MPs increased the sensitivity of H22 cells to drugs. H22 tumour cells were with or without the pretreatment of MPs and then incubated with different concentrations of MTX. After 6 h, the cells were washed and continued another 16 h culture. Apoptosis was determined by flow cytometry. Ten thousand events were collected for this analysis. Representative FACS profiles are shown on the left and the combined data from four reproducible experiments are shown on the right. Bars correspond to mean±s.d. *P<0.05, compared with control. Figure 6: MPs enhance tumour cell susceptibility to chemotherapy. ( a ) MPs decreased the efflux of drugs in H22 cells. H22 tumour cells were incubated with H22 cell-derived MPs for 12 h, then treated with 1 μg ml −1 doxorubicin. After 6 h, the supernatant was replaced with the fresh medium for another 6 h culture. The drug efflux by tumour cells was evaluated by flow cytometry and presented as the decrease of MFI. Data were combined from four reproducible experiments. Bars correspond to mean±s.d. ( b ) MPs increased the sensitivity of H22 cells to drugs. H22 tumour cells were with or without the pretreatment of MPs and then incubated with different concentrations of MTX. After 6 h, the cells were washed and continued another 16 h culture. Apoptosis was determined by flow cytometry. Ten thousand events were collected for this analysis. Representative FACS profiles are shown on the left and the combined data from four reproducible experiments are shown on the right. Bars correspond to mean±s.d. * P <0.05, compared with control. Full size image MPs deliver drugs to solid tumour via intravenous injection Although MPs were shown to effectively deliver drugs to local peritoneal tumours, it still remained to explore whether MPs were capable of delivering chemotherapeutic drugs to solid tumours. For this purpose, mice were subcutaneously inoculated with H22 cells. When tumour growth reached 5 × 5 mm 2 in size (5 days), mice were treated with MTX-packaged MPs via tail vein injection. After 7 days continuous injections, tumour growth was shown to be suppressed, compared with the control groups ( Fig. 7a ). Moreover, PKH26-conjugated MPs were i.v. injected to H22 tumour-bearing mice, and tumour was removed for fluorescence detection 4 h later. We found that MPs could be selectively recruited to the tumour site ( Fig. 7b ), suggesting that MPs may deliver chemotherapeutic drugs to solid tumours via the circulatory system. We also evaluated the influence of circulating MPs on coagulation. The pro-coagulant state of the mice was assessed after injection of MPs at different time points. We found that the prothrombin time, activated partial thromboplastin time and fibrinogen were not altered by MP injection ( Supplementary Fig. S13 ). 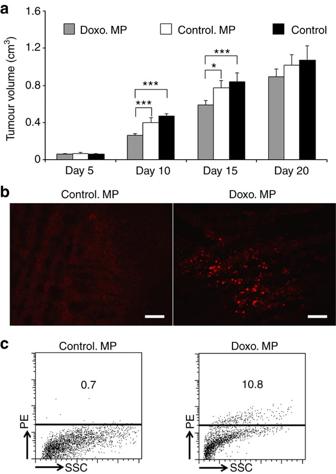Figure 7: Intravenouslyly injected MPs deliver chemotherapeutic drugs to solid tumours. (a) BALB/c mice (n=8) were inoculated with 2.5 × 105H22 cells subcutaneously. MPs-loaded doxorubicin were injected i.v. daily for 7 days, when tumour reached 5 × 5 mm2in size. Tumour growth was monitored (V=ab2/2). Data are representative of three independent experiments. Bars correspond to mean±s.d. *P<0.05; ***P<0.001. (b,c) MPs are accumulated in solid tumour site after i.v. injection. PKH26 (red)-conjugated MPs were injected to H22 subcutaneous tumour-bearing mice. After 4 h, tumour tissues were used for the analysis by fluorescence microscope (b). Scale bar, 100 μm. Ten thousand isolated tumour cells were collected for flow cytometric analysis of PKH26-positive population (c). Figure 7: Intravenouslyly injected MPs deliver chemotherapeutic drugs to solid tumours. ( a ) BALB/c mice ( n =8) were inoculated with 2.5 × 10 5 H22 cells subcutaneously. MPs-loaded doxorubicin were injected i.v. daily for 7 days, when tumour reached 5 × 5 mm 2 in size. Tumour growth was monitored ( V = ab 2 /2). Data are representative of three independent experiments. Bars correspond to mean±s.d. * P <0.05; *** P <0.001. ( b , c ) MPs are accumulated in solid tumour site after i.v. injection. PKH26 (red)-conjugated MPs were injected to H22 subcutaneous tumour-bearing mice. After 4 h, tumour tissues were used for the analysis by fluorescence microscope ( b ). Scale bar, 100 μm. Ten thousand isolated tumour cells were collected for flow cytometric analysis of PKH26-positive population ( c ). Full size image Artificial nanoparticles, such as liposome-packaging drugs, may have similar drug effects as tumour cell-derived MPs. MPs, derived from 1 mg ml −1 paclitaxel-treated 5 × 10 6 H22 tumour cells, and 60 μg liposome–paclitaxel generated a comparable cytotoxicity to H22 cells ( Supplementary Fig. S14 ). However, a tenfold increase in dosage applied in vivo resulted in different influences on mice weight. Six hundred micrograms liposome–paclitaxel caused a marked weight loss. Even 300 μg also negatively affected mice weight ( Supplementary Fig. S14 ). According to these results, 10-time MPs or 300 μg liposome–paclitaxel were i.v. injected to H22 tumour-bearing mice once per day for 7 days. Although the liposome–paclitaxel treatment inhibited tumour growth, the injection of MPs resulted in higher treatment efficiency ( Supplementary Fig. S14 ). Actin filaments affect the release and uptake of MPs To better understand drug-packaging MP-mediated tumour cell killing, the mechanism involved in tumour cell release and uptake of MPs was investigated. The cytoskeleton has important roles in cellular endocytosis and exocytosis [23] , [24] , [25] , [26] , leading to the possible requirement of cytoskeletal proteins for the release and uptake of MPs by tumour cells. When H22 cells were treated with cytochalasin D, an inhibitor of F-actin polymerization, actin filament formation was inhibited, resulting in decreased MP release, induced by ultraviolet irradiation ( Fig. 8a ). Furthermore, when H22 cells were treated with blebbistatin, the inhibition of actin filament motility also led to decreased MP release ( Fig. 8a ). When PKH-26-stained H22 cells, after treatment with cytochalasin D or blebbistatin, were incubated with CFSE-labelled MPs, to determine the uptake of MPs by tumour cells, an unexpected increase in the uptake of MPs by H22 tumour cells were found ( Fig. 8b ). Similar results were obtained from A2780 tumour cells. It is perhaps safe, therefore, to conclude from these findings that myosin II-triggered, actin filament-generated tension might mediate the release of MPs by tumour cells, whereas a soft microfilament cytoskeleton is perhaps more suitable for MP uptake. Whether this uptake is mediated through endocytosis was also investigated. The endo/lyosome tracker was used to merge the fluorescence of MPs. The result, however, did not show colocalization ( Supplementary Fig. S15 ). In parallel, the endoplasmic reticulum tracker and Golgi tracker were also used for the detection. Similarly, MPs appeared not to interact with endoplasmic reticulum or Golgi ( Supplementary Fig. S15 ). These data suggest that tumour cells take up MPs independent of endocytosis. 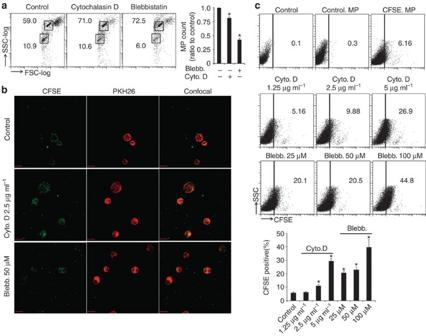Figure 8: Actin filaments are involved in release and uptake of MPs. (a) Actin filaments were required for the release of MPs. H22 cells were incubated with cytochalasin D or blebbistatin. After 5 h, cells were washed and irradiated with ultraviolet B. After 24 h, MPs in the supernatants were isolated and counted by flow cytometry with polystyrene Latex beads (3 μm) as standard (left). The dots in the upper and lower box were generated from standard beads (3 μm) and MPs, respectively. The right shown was the combined reproducible data (n=4). Bars correspond to mean±s.d. *P<0.05, compared with control group. (b,c) PKH-26 (red)-stained H22 tumour cells were treated with or without different concentration of cytochalasin D or blebbistatin for 5 h, and after the drugs were washed away cells were incubated with CFSE (green)-labelled MPs. After 16 h, cells were harvested and observed under confocal microscope (b) or analysed by flow cytometry (c). Scale bar, 10 μm. Data are representative of three reproducible independent experiments. Bars correspond to mean±s.d. *P<0.01, compared with control group. In this figure, 10,000–30,000 events were collected for flow cytometric analysis. Figure 8: Actin filaments are involved in release and uptake of MPs. ( a ) Actin filaments were required for the release of MPs. H22 cells were incubated with cytochalasin D or blebbistatin. After 5 h, cells were washed and irradiated with ultraviolet B. After 24 h, MPs in the supernatants were isolated and counted by flow cytometry with polystyrene Latex beads (3 μm) as standard (left). The dots in the upper and lower box were generated from standard beads (3 μm) and MPs, respectively. The right shown was the combined reproducible data ( n =4). Bars correspond to mean±s.d. * P <0.05, compared with control group. ( b , c ) PKH-26 (red)-stained H22 tumour cells were treated with or without different concentration of cytochalasin D or blebbistatin for 5 h, and after the drugs were washed away cells were incubated with CFSE (green)-labelled MPs. After 16 h, cells were harvested and observed under confocal microscope ( b ) or analysed by flow cytometry ( c ). Scale bar, 10 μm. Data are representative of three reproducible independent experiments. Bars correspond to mean±s.d. * P <0.01, compared with control group. In this figure, 10,000–30,000 events were collected for flow cytometric analysis. Full size image The biggest limitation of anticancer chemotherapy lies in its adverse effects [27] , [28] . To resolve this problem, innovative approaches to deliver chemotherapeutic agents are needed. As the carrier to deliver drugs, MPs have unique advantages: first, MPs are formed from cellular membranes, making them therefore much safer and self-friendlier; second, the preparation of drug-packaging MPs are very simple and easily manipulated; and third, packaging MPs with drugs is a general process and not restricted by physicochemical properties of drugs. The data gathered in this study reveal another critical feature of MP delivery. The use of MPs for the packaging and delivery of chemotherapeutic drugs reduces much of the toxicity of such drugs. The reasons for this advantage may be multiple and not reducible to one simple explanation. Physiological capillary gaps are around 5–8 nm (ref. 29 ), which prevents 100–1,000 nm MPs from reaching normal tissues and causing damage. Moreover, MPs were found to be very stable and resistant to detergent Triton X-100 consistent with previous reports that lipid rafts might be the main membrane component of MPs [30] , [31] . However, more important for the purposes of this paper it promises simple effective storage of drugs and innocuous therapeutic interventions in dealing with tumours. Therefore, MPs may well represent a new and more patient friendly approach to deliver chemotherapeutic agents. Recent studies highlight that lymphocytes, neutrophils, NK cells and even tumour cells can live temporarily within tumour cells, a phenomenon called cell cannibalism or cell-eat-cell [32] , [33] . Therefore, it might be easy for tumour cells to take up MPs, even though the detailed mechanisms remain unclear. Intriguingly, this uptake is not mediated through endocytosis pathways, so that how MPs release chemotherapeutic molecules within tumour cells is still elusive. Furthermore, regardless of the homology between MPs and tumour cells, it is inevitable that MPs will be taken up by phagocytes, such as macrophages [15] , [34] , [35] . This, however, might actually be beneficial to cancer treatment, because tumour-associated macrophages have very important roles in tumour development by promoting neoangiogenesis, remodelling tumour microenvironment and dampening the immune response to tumours [36] , [37] , [38] , [39] . In this study, we observed that peritoneal macrophages took up drug-packaging MPs and then died. Whether and how such killing of tumour-associated macrophages synergizes with the killing of tumour cells by drug-packaging MPs to generate better therapeutic effects is currently under study. Peritoneal neoplasia can originate de novo from the peritoneal tissues as primary tumours [40] , [41] . However, in most cases, it is derived from the invasion of adjacent tumours or metastasis of remote tumours [42] , [43] . Although the peritoneal metastasis of colon, liver and pancreatic cancers is not common, clinical ovarian cancer is almost always accompanied by peritoneal metastasis when diagnosed [44] , [45] . In the present study, drug-packaging MPs were used to treat peritoneal cancers inoculated with either murine hepatocarcinoma or human ovarian cancer tumour cells. Striking therapeutic efficiencies were observed, in the form of total inhibition of tumour growth in part tumour-bearing mice, even when the packaged drug quantity and the doses of administered MPs were not optimal. H22 cells grow very quickly in the peritoneal cavity, which results in the observed ascites on day 5 and peaked on day 8 or 9, then maintaining this level owing to space limitations. The single MTX treatment has therapeutic effect only at the beginning, which delays the visible ascites 1 or 2 days, but the ascites came back soon. This very malignant tumour model is chosen in order to emphasize the efficiency of MP-based therapeutics. On the other hand, the difference between normal (5–8 nm) and tumour capillary permeability (100–780 nm) [29] , [46] , [47] implies that MPs might be used to deliver drugs to solid tumours by blood flow. This study additionally provides evidence that the delivery of chemotherapeutic to solid tumours by MPs is feasible via direct intravenous injections. Although MPs were found to migrate to the tumour site and be taken up by tumour cells after i.v. injection, the complex and intricate dynamics of such drug-packaging MPs in the blood stream still remains to be elucidated. Previous works by Jain and colleagues [46] have demonstrated that the increases in tumour vascular permeability form the basis for nanoparticle extravasation and drug delivery. Recently, works by Dass and colleagues [48] have shown that chitosan-based delivery systems are efficient for cancer therapy. Along with these studies, current advances in nanotechnology have produced synthetic nanoparticles to encapsulate and release a pre-programmed diversity of therapeutic measures against cancers [1] , [2] , [4] , [49] , [50] , [51] . These artificial materials are, however, known to often induce immune responses, leading to minor or even serious adverse effects [3] , [4] , [5] , [6] , [7] . Furthermore, nanoparticles range in size from 20 and 50 nm (refs 2 , 49 ), limiting the number of chemotherapeutic molecules that can be packaged. Besides, polymeric micelle systems generally suffer from poor water-soluble drug-incorporation efficiencies. This is because of the small size and hence large surface area of drugs, which promote drug loss into the aqueous phase during particle formation. In contrast, water-soluble drugs are ideal for MPs packaging. As natural self-components, MPs do not induce autoimmunity and range in size from 100 to 1,000 nm, guaranteeing the efficacy of MPs as therapeutic vector to package needed and sufficient enough therapeutic agents. More importantly, this present study indicates that MPs, as natural biomaterials, possess unique merits, such as domino-like killings, where drug-packaging MPs can trigger the formation of new drug-packaging MPs after entering into tumour cells, and inhibiting the efflux of chemotherapeutic drug by tumour cells. The latter has important implications for cancer therapy with regard to multidrug resistance [52] , [53] . This study does not identify or map the exact pathways through which MPs impede the efflux of chemotherapeutic drugs. However, one possibility is that, owing to their compatibility to tumour cell membranes, MP membranes might be integrated into tumour cell membranes, resulting in the blockage of drug-efflux pumps. Further study is required to clarify this. In summary, the data in this study clearly show that tumour cell-derived MPs, by virtue of their biological formation and subsequent biochemical features, can be used as a carrier to deliver therapeutic agents to tumour cells, leading to effective tumour cell killing with reduced adverse effects. This study may open a new aspect of MP biology and may have discovered a new way for chemotherapeutic drug delivery in cancer therapy. Mice and cell lines Female BALB/c and BALB/c-SCID mice, 6- to 8-week-old, were purchased from Centre of Medical Experimental Animals of Hubei Province (Wuhan, China) for studies approved by the Animal Care and Use Committee of Tongji Medical College. Murine hepatocarcinoma cell line H22 and human ovarian cancer cell line A2780 were purchased from China Centre for Type Culture Collection (CCTCC, Wuhan, China), and cultured according to the guidelines given. Generation and isolation of MPs Tumour cells were treated with chemotherapeutic drug MTX, hydroxyl camptothecin or cisplatin, and then exposed to ultraviolet irradiation (UBV, 300 J m −2 ) for 1 h. After 12 h, supernatants were used for MP isolation as described before [16] , [17] . Briefly, supernatants were first centrifuged for 10 min at 600 g to get rid of cells and then centrifuged for 2 min at 14,000 g to remove debris. At last, the supernatant was further centrifuged for 60 min at 14,000 g to pellet MPs. The pellets were washed three times and resuspended in culture medium for the following experiments. MP counting A flow cytometry-based method was used to count the number of MPs. After centrifugation, the MPs were suspended with PBS that was prefiltered through 0.1 μm filter and passed through 1 μm filter to further exclude background noise or nonspecific events. The MPs mixed evenly with 3 μm latex beads (LB-30, Sigma, St Louis, MO) with a known number. For flow cytometric analysis, 0.8 μm deep-blue dyed-latex beads (L1398, Sigma) were first used for gating and voltage adjustment, as such beads are fluorescent and can be detected on FL4 channel. When the mixture was analysed by flow cytometry, each LB30 bead formed a dot in the gate of the large-size population. If 10,000 counts of LB30 were collected, the number of MP can be calculated with formula: N =10,000 × (MP percentage/LB30 percentage). Transmission electron microscope MPs were passed through 1 μm filter and fixed at room temperature for 60 min with 4% paraformaldehyde in 0.01 M PBS. After washing with PBS, the preparations were postfixed in 1% OsO4 (Taab) for 30 min. After rinsing with distilled water, the pellets were dehydrated in graded ethanol, including block staining with 1% uranylacetate in 50% ethanol for 30 min, and embedded in Taab. After overnight polymerization at 60 °C and sectioning for EM, the ultrathin sections were analysed with a JEM1010 electron microscope (JEOL, Japan). Assay of MPs packaging chemotherapeutic agents Doxorubicin, a red-fluorescent chemotherapeutic drug, was used to treat H22 or A2780 tumour cells. The released MPs were isolated and observed under a two-photon fluorescent microscope (LSM 710 and ConfoCor 3 systems, Carl Zeiss, Germany) to confirm the formation of MPs packaging chemotherapeutic agents. High-performance liquid chromatography The concentration of chemotherapeutic drug in MPs was measured by HPLC. Briefly, H22 tumour cell-derived, doxorubicin-packaging MPs were processed by lysis buffer, proteinase K, phenylmethylsulphonyl fluoride and DNase I according to previous description [54] . The HPLC system consisted of a 1525 Binary HPLC Pump, a 717 Plus Autosampler and a 2475 Multi-Wavelength Fluorescence Detector (Waters Corporation, Milford, CT). Chromatography was performed on a column (4.6 × 150 mm 2 , particle size 5 μm). The effluents were monitored at an excitation wave length of 480 nm and an emission wave length of 560 nm at 40 °C. Detection and integration of chromatographic peaks was performed using Empower 2 software (Waters Corporation). Cytotoxicity assay of drug-packaging MPs Drug-packaging MPs were prepared and added to the cultured tumour cells. The cells were observed under a microscope at different time points. In some cases, cells were collected and stained with annexin V and propidium iodide for apoptosis detection by a flow cytometer. Labelling of MPs Isolated MPs were labelled with a red-fluorescent cell linker (PKH26, Sigma) according to the manufacturer’s protocol. Flow cytometry A BDTM LSR II flow cytometer (BD) was used to do the flow cytometric analysis of the MPs in samples. The instrument settings and MP gating were adopted from previous works [55] . Samples were diluted in 1:30 with 1.2-μm pore size membrane-filtered PBS in order to reduce background event numbers. A microbead of 3 μm in diameter (Sigma-Aldrich) was used to select optimal instrument settings and MP gate. Total event counts of MPs were determined within the MP gate. Animal model and MP treatment protocol 1 × 10 5 H22 murine hepatocarcinoma tumour cells (BALB/c background) were i.p. injected into BALB/c mice. Seven days later, the growth of H22 tumour cells formed hepatocarcinoma ascites. To treat this peritoneal tumour, 2 mg MTX was added to 2 × 10 7 H22 tumour cells in 2 ml culture medium and the prepared MTX-packaging MPs were then administered to one mouse per packaged MPs. On day 2 after H22 tumour cell inoculation, mice were received MTX-packaging MPs by i.p. injection once per day for 5 days. For the human ovarian cancer murine peritoneal model, BALB/c-SCID mice were i.p. injected with 5 × 10 6 A2780 human ovarian cancer tumour cells. On day 2 after the inoculation, MPs generated from 2 × 10 7 A2780 cells treated with cisplatin (300 μg ml −1 ) were i.p. injected to mouse once per day for 5 days. After day 14, an additional treatment was administered once per day for 5 days. On day 30, half the mice were killed for tumour detection and the left mice were fed for the long-term survival study. In selected cases, drug-packaging MPs and paclitaxel–liposome were i.v. injected to mice. Paclitaxel–liposome, which was approved by the State Food and Drug Administration of China (No. H20030357), was purchased from Nanjing Si Ke Pharmaceutical Co., Ltd. (Nanjing, China) as freeze-dried powder in glass vials containing 30 mg of active drug. Hoechst 33342 uptake assay Isolated MPs treated with or without 0.5% Triton X-100 were incubated with Hoechst 33342 for 12 h. MPs were isolated again resuspended in 30 μl PBS buffer. Suspensions were smeared on a glass slide and photographed under a fluorescence microscope. Assay of tumour cells taking up MPs in vitro CFSE-labelled H22 cells treated with UBV irradiation (300 J m −2 ) were cultured for 24 h. MPs were isolated from the supernatant, and then incubated with PKH 26-stained H22 cells for 20 h. Cells were observed by two-photon confocal microscope or analysed by flow cytometry. Peritoneal H22 tumour cell isolation 3 × 10 5 H22 tumour cells were i.p. injected into BALB/c mice. Peritoneal tumour cells were isolated at different time points. Briefly, peritoneal cells were harvested and centrifugated. After lysis of RBC, cells were incubated on ice for 20 min and then spun down at 500 revolutions per minute. for 1 min. This process was repeated twice and the spun cells were further incubated for 2 h to get rid of adhesive cells. The cells left were used as H22 tumour cells. Mouse primary hepatocyte isolation Mouse primary hepatocytes were isolated from BALB/c mice using a two-step collagenase perfusion as described previously [56] . The viable hepatocyte population was further purified by a Percoll gradient centrifugation [57] . Hepatocytes were resuspended and seeded onto collagen-coated plates at 2 × 10 5 cells per well in a 6-well plate in Williams’ E medium (Invitrogen) with 10% FBS, insulin (0.5 μg ml −1 , Sigma), dexamethasone (50 nM, Sigma), streptomycin (0.1 mg ml −1 ) and penicillin G (100 U ml −1 ) at 37 °C and under 5% CO 2 . Assaying second and third generations of MPs H22 tumour cells were treated with 250 μg ml −1 doxorubicin to prepare the first generation of MPs. Such doxorubicin-packaging MPs were incubated with fresh H22 tumour cells. After 6 h, cells were washed and irradiated with UBV (300 J m −2 ). After another 24 h, the released MPs packaging doxorubicin were detected with two-photon confocal microscope or flow cytometry and called the second generation of MPs. In the same way, the third generation of MPs were prepared. Statistics analysis Results were expressed as mean values±s.d. and interpreted by repeated-measure analysis of variance or Kaplan–Meier analysis. Differences were considered to be statistically significant when the P -value was <0.05. How to cite this article: Tang, K. et al . Delivery of chemotherapeutic drugs in tumour cell-derived microparticles. Nat. Commun. 3:1282 doi: 10.1038/ncomms2282 (2012).